Polyoxometalate-mediated electron transfer–oxygen transfer oxidation of cellulose and hemicellulose to synthesis gas Terrestrial plants contain ~70% hemicellulose and cellulose that are a significant renewable bioresource with potential as an alternative to petroleum feedstock for carbon-based fuels. The efficient and selective deconstruction of carbohydrates to their basic components, carbon monoxide and hydrogen, so called synthesis gas, is an important key step towards the realization of this potential, because the formation of liquid hydrocarbon fuels from synthesis gas are known technologies. Here we show that by using a polyoxometalate as an electron transfer–oxygen transfer catalyst, carbon monoxide is formed by cleavage of all the carbon–carbon bonds through dehydration of initially formed formic acid. In this oxidation–reduction reaction, the hydrogen atoms are stored on the polyoxometalate as protons and electrons, and can be electrochemically released from the polyoxometalate as hydrogen. Together, synthesis gas is formed. In a hydrogen economy scenario, this method can also be used to convert carbon monoxide to hydrogen. Environmental concerns and decreasing amounts of fossil fuels, especially oil, is leading to the development of renewable resources for liquid fuels and feedstock for petrochemicals. Solar energy and solar fuels have been touted as the ultimate, indefatigable sources of energy, but the storage of sunlight and its use in a practical way remains a major challenge of our generation. In this context, the storage of solar energy in terrestrial biomass takes advantage of natural photosynthetic pathways and further biosynthetic reactions using CO 2 and H 2 O as carbon and hydrogen atom sources. Typically, biomass contains 35–50% cellulose, 20–35% hemicellulose and 10–25% lignin. An emerging field is biorefining of biomass and processes, including catalytic hydrolysis, solvolysis, liquefaction, pyrolysis, gasification, hydrogenolysis and hydrogenation, are all being considered [1] , [2] . The transformation of cellulose to D -glucose, its sole component, and then to ethanol to be used as a biofuel by fermentation is perhaps the most developed technology; however, the failure of simple acids to hydrolyse cellulose selectively [3] remains a problem that requires the use of more expensive cellusomes [4] . The hydrolysis/fermentation approach also has the disadvantage that hemicellulose and its major hydrolysis product, D -xylose, still cannot be used to form ethanol. On the other hand, cellulose/hemicellulose hydrolysis has been suggested as a route to platform chemicals such as sugars, formic acid, levulinic acid and hydroxymethylfurfuraldehyde among others [5] , [6] . Other efforts have been made to convert cellulose or cellulose-derived materials to hydrocarbons [7] , [8] , [9] , hydrogen [10] , [11] and furans [12] . Despite the aforementioned advances, reaction selectivity is typically low and process schemes are quite complicated [5] , [6] , [7] , [8] , [9] , [10] , [11] , [12] . Here we describe a two-step, one-pot conversion of both cellulose and hemicellulose to synthesis gas, CO and H 2 with high selectivity at mild conditions combining an anaerobic oxidation with the electrochemical release of H 2 . Synthesis gas is a known industrial commodity that can be used in various ways, including for the formation of hydrocarbon fuels via the Fischer–Tropsch process [13] , the synthesis of methanol [14] and in transformations such as hydroformylation [15] . We also demonstrate that synthesis gas can be transformed to H 2 via a variant water gas shift reaction [16] , using the same catalytic system. Mechanism of the carbon–carbon bond cleavage The transformation of cellulose and hemicellulose polysaccharides, (C n H 2 n O n ) m where n =6 for D -glucose and n =5 for D -xylose to synthesis gas is based on our previous studies that showed that the H 5 PV 2 Mo 10 O 40 polyoxometalate catalyses reaction by an electron transfer–oxygen transfer-type mechanism [17] , [18] . In such a generic reaction, oxygen atoms are transferred from the polyoxometalate to the organic substrate; the polyoxometalate is reduced. Typically, in a second step molecular oxygen is used to reoxidize the polyoxometalate. In particular, H 5 PV 2 Mo 10 O 40 was found to catalyse the carbon–carbon bond cleavage of vicinal diols and primary alcohols by an oxygen insertion reaction into the carbon–carbon bond [19] . As D -glucose has both these moieties, a predictive analysis shows that it could yield 5 equivalents of HCOOH, 1 equivalent of HCHO and 6 equivalents of reduced polyoxometalate, H 7 PV IV 2 Mo 10 O 40 according to a series of reactions presented in Fig. 1 . 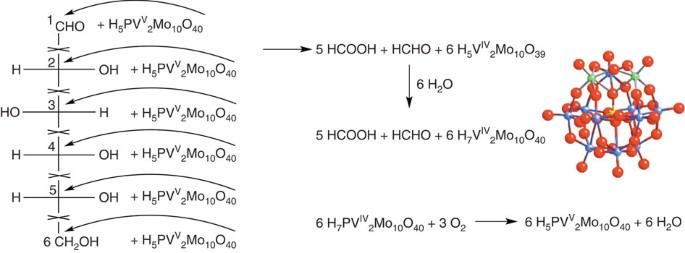Figure 1: The predicted oxidative cleavage ofD-glucose. The reaction of glucose, presented as a Fisher projection for simplicity, with 6 equivalents of H5PVV2Mo10O40shows the carbon–carbon bond cleavage reactions. The molecular structure of the 1,2 isomer of H5PVV2Mo10O40is shown in the insert; P: yellow, Mo: blue, V: green and O: red. Other isomers have similar reactivity17. Figure 1: The predicted oxidative cleavage of D -glucose. The reaction of glucose, presented as a Fisher projection for simplicity, with 6 equivalents of H 5 PV V 2 Mo 10 O 40 shows the carbon–carbon bond cleavage reactions. The molecular structure of the 1,2 isomer of H 5 PV V 2 Mo 10 O 40 is shown in the insert; P: yellow, Mo: blue, V: green and O: red. Other isomers have similar reactivity [17] . Full size image The reaction is surmised to ideally proceed via an oxygen atom insertion from the polyoxometalate accompanied by carbon–carbon bond cleavage to yield formic acid (HCOOH) from the C-1 to C-5 carbon atoms and formaldehyde (HCHO) from the C-6 carbon atom. The deoxygenated and reduced polyoxometalate, H 5 PV IV 2 Mo 10 O 39 reacts with H 2 O to yield H 7 PV IV 2 Mo 10 O 40 . If the reaction is carried out in the presence of O 2 , its reaction with H 7 PV IV 2 Mo 10 O 40 will yield H 5 PV V 2 Mo 10 O 40 and H 2 O as shown in Fig. 1 . Thus, the oxidation of D -glucose was studied under such conditions using 1:1 methanol/water as a solvent, which allowed reaction at low O 2 pressure. Essentially quantitative conversions of D -glucose were obtained according to Fig. 2 , where the presence of methanol in the acidic reaction medium leads to further partial ester, hemiacetal and acetal formation. Methanol is oxidized only in trace amounts under these conditions. 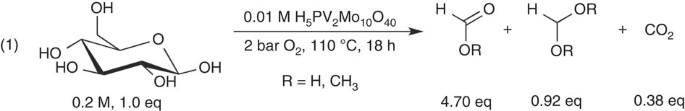Figure 2: Aerobic oxidation ofD-glucose. D-glucose (100 mg, 0.56 mmol), H5PV2Mo10O40·32H2O (88 mg, 0.038 mmol), 3 ml of a (1:1) mixture of CD3OD and D2O were dissolved in a 50-ml glass pressure tube. Reactions were carried at 2 bar O2at 110 °C for 18 h. Figure 2: Aerobic oxidation of D -glucose. D -glucose (100 mg, 0.56 mmol), H 5 PV 2 Mo 10 O 40 ·32H 2 O (88 mg, 0.038 mmol), 3 ml of a (1:1) mixture of CD 3 OD and D 2 O were dissolved in a 50-ml glass pressure tube. Reactions were carried at 2 bar O 2 at 110 °C for 18 h. Full size image The results showed a good correlation with the expected theoretical results presented in Fig. 1 . There was only slight overoxidation to CO 2 . To further delineate and support the proposed reaction scheme, reactions were carried out with isotopically labelled carbon-13 glucose derivatives. A reaction using 13 C 6 H 12 O 6 revealed peaks in the 13 C NMR spectrum at 165.3, 164.1, 97.0, 89.7 and 82.2 p.p.m. assignable to H C OOH, H C OOCH 3 , C H 2 (OCH 3 ) 2 , C H 2 (OH)(OCH 3 ) and C H 2 (OH) 2 , respectively ( Supplementary Fig. 1 ). Six individual reactions carried out with 13 C 12 C 5 H 12 O 6 where D -glucose was labelled at the C-1 to C-6 carbon atoms showed that most of the formaldehyde derivatives originated from the C-6 carbon atom with a small amount originating from the C-1 carbon atom. The C-2 to C-5 carbon atoms yielded formic acid and its methyl ester only and the C-1 carbon atom likewise yielded mostly, >95%, these products. The labelling experiments also support the reaction presented in Fig. 1 . Interestingly, aliquots taken from the gas phase and analysed by gas chromatography (GC)–mass spectrometry showed 13 CO 2 was formed mostly from the C-5 carbon atom. This suggests that the hemiacetal present in the pyranose conformation leads to more formation of CO 2 . Finally, a stoichiometric reaction where one equivalent polyoxometalate per carbon atom was reacted under anaerobic conditions yielded reduced polyoxometalate and showed 12±0.2 electron equivalents per equivalent D -glucose as expected from the reaction stoichiometry ( Fig. 1 ). Other saccharides reacted similarly ( Supplementary Table 1 ). Formation of synthesis gas from cellulose and hemicelluloses It has been shown that H 5 PV 2 Mo 10 O 40 can convert carbohydrates such as hemicellulose in water under rather high O 2 pressures (30 bar) to formic acid in only a 50% yield with co-formation of 50% CO 2 but cellulose reacted in only low yields [20] , [21] . Vanadium oxide and sodium vanadate gave similar results [22] , [23] . The maximum yield of formic acid is around 50% for hemicellulose and around only 7% for cellulose in the presence of O 2 (refs 20 , 21 , 22 , 23 ). Formic acid has been suggested as an energy carrier or chemical intermediate in numerous scenarios. It can be transformed to H 2 and CO 2 (refs 24 , 25 , 26 ), or acid-catalysed dehydration of formic acid to CO and H 2 O can be contemplated [27] . Notably, formic acid alone cannot yield both CO and H 2 . Analysis of the H 5 PV 2 Mo 10 O 40 electron transfer–oxygen transfer oxidation of glucose, Fig. 1 , shows that initially hydrogen atoms are ‘stored’ on polyoxometalate as electrons and protons, which under O 2 leads to formation of H 2 O. Reoxidation of the polyoxometalate under anaerobic conditions will prevent H 2 O formation and allow the formation of H 2 . As a saccharide unit such as D -glucose, C 6 H 12 O 6 , has the theoretical potential to yield 6 equivalents of both CO and H 2 , three major questions were asked: (1) can the electron transfer–oxygen transfer oxidation reactivity found for D -glucose be realized also for polysaccharides, specifically for hemicellulose and cellulose; (2) how can the originally formed formic acid and formaldehyde be converted to CO; and (3) how can H 2 be formed? Initial experiments showed that formic acid could be quantitatively converted to 99% CO and 1% CO 2 in concentrated H 2 SO 4 (1 ml formic acid, 100 mg 98% H 2 SO 4 , 100 °C, 8 h). Not surprisingly, the addition of water proportionally reduced the reaction conversion but did not affect selectivity. Based on this observation, cellulose and hemicellulose were reacted with H 5 PV 2 Mo 10 O 40 in concentrated H 2 SO 4 under anaerobic conditions as shown in Fig. 3 . The cellulose used was microcrystalline powder from natural wood pulp and the hemicellulose was xylan from beechwood. Both were used without any pre-treatment. The reactions were carried out by mixing 100 mg polysaccharide, 7.80 g (3.3 mmol) H 5 PV 2 Mo 10 O 40 ·32H 2 O in 8 ml 98% H 2 SO 4 at 70 °C for 5 h under N 2 . As the polyoxometalate is solvated by 32 water molecules, the concentration of H 2 SO 4 during the reaction is ~80 vol%. There was complete conversion for both cellulose and hemicellulose as verified by the absence of any 1 H NMR signals when the reaction was carried out in D 2 SO 4 . Notably, there was no observable char formation ( Supplementary Fig. 2 ). Analysis of the gas phase by GC with a thermal conductivity detector (GC-TCD) showed the formation of only CO and CO 2 in a ratio that was on the average 65±3:35±3 over five experiments. In addition, quantitative analysis using the GC-TCD with N 2 as the internal standard showed quantitative formation, that is, 97±4% of CO and CO 2 . Other acids were also suitable for this reaction ( Supplementary Table 2 ). 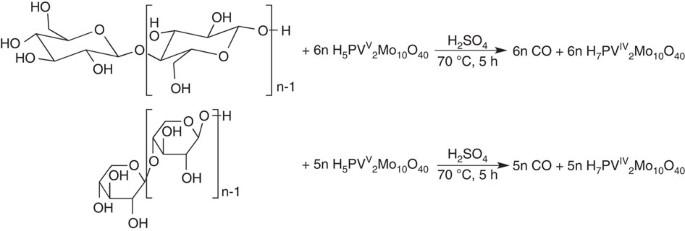Figure 3: Anaerobic oxidation of cellulose and xylan hemicelluloses. The reaction shows the general transformation of cellulose and xylan hemicellulose in H2SO4with H5PV2Mo10O40. Figure 3: Anaerobic oxidation of cellulose and xylan hemicelluloses. The reaction shows the general transformation of cellulose and xylan hemicellulose in H 2 SO 4 with H 5 PV 2 Mo 10 O 40 . Full size image The reason for the formation of CO 2 under anaerobic conditions was not immediately clear. As after only 30 min the CO:CO 2 ratio was 5:1, it was suspected that CO was being oxidized also by an electron transfer–oxygen transfer mechanism by H 5 PV 2 Mo 10 O 40 according to equation 1 below [27] . The observation that CO was partially oxidized further after it was initially formed also allowed some further mechanistic insight into the oxidation of saccharides by H 5 PV 2 Mo 10 O 40 . Thus, six individual reactions were carried out with 13 C 12 C 5 H 12 O 6 where D -glucose was labelled individually at the C-1 to C-6 carbon atoms (10 mg (0.056 mmol) D -glucose ( 13 C 12 C 5 H 12 O 6 ), 0.78 g (0.33 mmol) H 5 PV 2 Mo 10 O 40 ·32H 2 O, 1 ml 98% H 2 SO 4 , 3 h, 70 °C, N 2 ). The results showing the 13 CO/ 13 CO 2 ratio for each of the six reactions are shown in Table 1 . Table 1 The 13 CO/ 13 CO 2 ratio observed in the oxidation of individually 13 C labelled D -glucose isomers*. Full size table Clearly, the results indicate that the C-5 and C-4 atoms yield the most CO 2 , leading to the conclusion that these positions were the first to be oxidized/dehydrated to CO. The C-5 hemiacetal in pyranose form of D -glucose and the adjacent C-4 appear to be most susceptible to oxidation with H 5 PV 2 Mo 10 O 40 . Interestingly, the aldehydic C-1 atom yielded less CO 2 than the primary C-6 atom consistent with the previously observed unusual reactivity of H 5 PV 2 Mo 10 O 40 with primary alcohols that gives C–C bond cleavage rather than oxidation at the primary alcohol [19] . Note that the pathway for the formation of CO from the C-6 atom could be directly from the initially formed formaldehyde or through formic acid. It seems likely to be that cellulose is oxidized in a similar way, although the question remains whether glycosidic bonds are initially hydrolysed or not. At the completion of the reaction, the original orange solution associated with oxidized H 5 PV V 2 Mo 10 O 40 turns deep blue. Titration with KMnO 4 showed an average over five experiments of 2.7±0.2 equivalent electrons per equivalent carbon atom. As vanadium is reduced before molybdenum [17] , [18] , reaction stoichiometry H 7 PV IV 2 Mo VI 10 O 40 and H 8 PV IV 2 Mo V Mo VI 9 O 40 are apparently present in the reaction mixture in a ~7:3 ratio. The cyclic voltammetry measurements of this reaction solution, 0.42 M H 5 PV 2 Mo 10 O 40 in H 2 SO 4 , reduced by 2.7 electrons, Fig. 4 (left), showed a redox potential of 0.4 V versus normal hydrogen electrode. Oxidation of 25–30% of the polyoxometalate at 0.6 V resulted in a change in the colour of the solution to a dark green and a shift of the redox potential to 0.05 V versus normal hydrogen electrode, Fig. 4 (right). From this, it would appear that first H 8 PV IV 2 Mo V Mo VI 9 O 40 is oxidized to H 7 PV IV 2 Mo VI 10 O 40 , which is then oxidized to H 5 PV V 2 Mo 10 O 40 . The exact reason for this change in redox potential is still uncertain but previous studies have shown that the degree of reduction of the polyoxometalate has structural implications, wherein different coordinatively unsaturated compounds are formed [18] . These different coordinatively unsaturated compounds are likely to have different redox potentials. Therefore, to form H 2 quantitatively the solution was oxidized using a Pt gauze electrode. Oxidation was at 0.6 V for 25–30% of the total number of coulombs needed and then the oxidation of the polyoxometalate was completed at 0.2 V. The total coulomb count gave the same average number of electrons as the KMnO 4 titration ( Supplementary Fig. 3 ). Hydrogen was collected and its quantitative formation verified by GC. 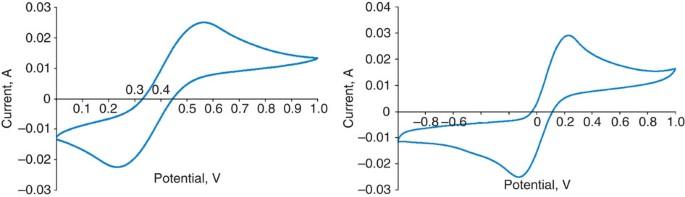Figure 4: Cyclic voltammograms of the reaction solution. Cyclic voltammogram of a reaction solution originally containing 0.42 M H5PV2Mo10O40in H2SO4. Pt was used as the working and counter electrode and the H+/H2couple catalysed by Pt was the reference. Scan rate: 200 mV s−1. Left: at the end of cellulose oxidation, which is 2.7 electrons/H5PV2Mo10O40. Right:after oxidation at 0.6 V and 25–30% oxidation of the polyoxometalate leaving 2.0 electrons/H5PV2Mo10O40. Figure 4: Cyclic voltammograms of the reaction solution. Cyclic voltammogram of a reaction solution originally containing 0.42 M H 5 PV 2 Mo 10 O 40 in H 2 SO 4 . Pt was used as the working and counter electrode and the H + /H 2 couple catalysed by Pt was the reference. Scan rate: 200 mV s −1 . Left: at the end of cellulose oxidation, which is 2.7 electrons/H 5 PV 2 Mo 10 O 40 . Right:after oxidation at 0.6 V and 25–30% oxidation of the polyoxometalate leaving 2.0 electrons/H 5 PV 2 Mo 10 O 40 . Full size image Water gas shift reaction As noted above, CO is partially oxidized to CO 2 in the absence of O 2 during the transformation of the carbohydrates. In the past, such a transformation has been carried out using a polyoxometalate together with a gold catalyst [28] . This leads to the possibility that H 5 PV 2 Mo 10 O 40 alone in a mineral acid could be used to carry out a water gas shift reaction at very low temperatures. In this context, such a water gas transformation is in itself an interesting alternative to the higher temperature water gas shift reaction presently practiced, because (1) it is thermodynamically more efficient at low temperature (Δ G r,g,25 °C =−5.8 kcal mol −1 although the Δ G r in H 2 SO 4 is unknown) and (ii) the separate catalytic CO 2 and electrochemical H 2 -forming steps obviate the necessity of separating CO 2 from H 2 . For example, in a glass pressure tube 2 bar of CO was reacted with 1.4 mmol H 5 PV 2 Mo 10 O 40 ·32H 2 O dissolved in 8 ml 80% aqueous H 2 SO 4 . After 5 h at 100 °C, complete conversion was attained and H 2 was released electrochemically as described above. A representation of the transformation of cellulose and hemicellulose using cellulose as a representative substrate is presented in Fig. 5 , where both the electron transfer–oxygen transfer oxidation of the carbohydrate and the oxidation of CO are shown along with the electrochemical oxidation of the electrons and protons initially stored on the polyoxometalate. 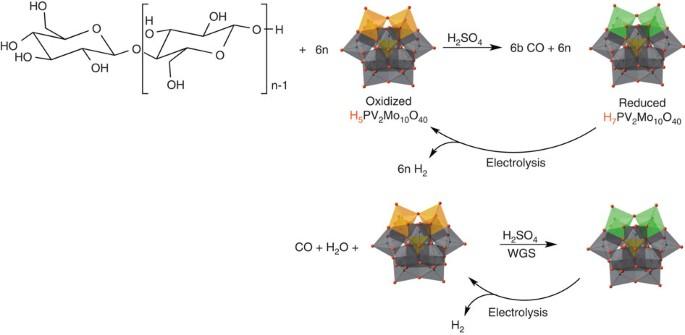Figure 5: Conversion of cellulose. The conversion of cellulose to CO and H2and the water gas shift of CO. Figure 5: Conversion of cellulose. The conversion of cellulose to CO and H 2 and the water gas shift of CO. Full size image Several summary points are notable. (1) This is the first reported use of concentrated sulphuric acid, an inexpensive industrial commodity, in a polyoxometalate-catalysed reaction that now allows the complete transformation of both cellulose and hemicellulose at mild reaction temperatures. The initially formed formic acid is formed in a high yield and then quantitatively dehydrated to CO. The electrochemical release of H 2 for the most part at a relatively low over-potential of 0.2 V allows the overall formation of synthesis gas, 1 equivalent of CO and H 2 per carbon atom. (2) The use of H 2 SO 4 has the added advantage that it significantly increases the rate of the electron transfer–oxygen transfer oxidation and is a convenient medium for the release of H 2 at low potentials. (3) Fast removal of the CO formed by purging the reaction mixture can prevent its further oxidation to CO 2 . However, if H 2 were the target, the complete conversion of CO by a water–gas shift reaction using this catalytic system can be used. In this way, 2 equivalents of H 2 can be formed per carbon atom in the polysaccharide. (4) The separate electrochemical release of H 2 can allow separate formation of H 2 and CO. (5) Importantly, after the formation of only gaseous products, the reaction solution, that is, H 5 PV 2 Mo 10 O 40 in H 2 SO 4 , can be recycled and reused without any additional treatment. Ten reaction cycles using cellulose as substrate showed no change in reactivity. In this context, it can be noted that we observed that vanadium oxide also can oxidize carbohydrates in H 2 SO 4 ; however, H 2 cannot be recovered electrochemically. The research presented herein could be the foundation for a new technology for the formation of synthesis gas from biomass. Purported advantages of the proposed concept are: (1) as solar energy and other sources (wind, geothermal and nuclear) are more simply transformed to electric power compared with their storage as a chemical fuel, the low-temperature electrochemical approach presented here has the potential for considerable total energy saving and (2) the synthesis gas yield can be significantly higher than what can be obtained with high-temperature steam reforming of biomass where the need to use O 2 from air leads to formation of CO 2 as the major product, which is not compensated by H 2 formation, and which require noble metal-based catalysts for quantitative conversions [29] . (3) The concept presented herein indicates a requirement of 1 mole equivalent of polyoxometalate per carbon atom; for example, 10 mg of cellulose per 780 mg polyoxometalate in a one-pot reaction. However, as the cellulose conversion is quantitative, all the products are gaseous and the catalyst is very stable under reaction conditions, in a perceived technological application using a continuous reaction mode carbohydrates can be fed and synthesis gas can be removed continuously with a fixed amount of catalyst. Materials Microcrystalline cellulose, hemicellulose and the other sugars were purchased from Sigma-Aldrich. Microcrystalline cellulose was from natural wood pulp and was of an unknown molecular weight. It was used without pre-treatment. Hemicellulose was xylan from beechwood and was used without any pre-treatment. The seven carbon-13-labelled glucose compounds, and CD 3 OD, D 2 O and D 2 SO 4 were purchased from Cambridge Isotope Laboratories. H 5 PV 2 Mo 10 O 40 ·32H 2 O was prepared by a known procedure [30] . Aerobic reactions Aerobic reactions in water/methanol were carried out by dissolving 100 mg saccharide or polysaccharide, 88 mg H 5 PV 2 Mo 10 O 40 ·32H 2 O (0.038 mmol) in 3 ml of a (1:1) mixture of CD 3 OD and D 2 O in a 50-ml glass pressure tube. Reactions were carried at 2 bar O 2 , 110 °C for 18 h. The amount of products formed, formic acid, methyl formate, dimethoxymethane, methoxymethanol and methanediol were calculated using 300 MHz 1 H NMR and ethanol as an external standard. As the peak for H 2 O (always present to some degree) partially overlapped with those of the formaldehyde derivatives, two drops of 35% HCl were added to shift the peak of water downfield. CO 2 and CO were determined by GC-TCD using a GowMac instrument with a 20′ × 1/8″ stainless steel column packed with molecular Sieve 5 Å in series with a 4′ × 1/8″ stainless steel column packed with HayeSep T. The carrier gas was Ar, column T =120 °C. Retention times for CO 2 was 4.5 min and for CO was 30.2 min. Supplementary Table 1 shows the results for a variety of saccharides and polysaccharides. Anaerobic reactions Anaerobic oxidation in concentrated (98%) sulphuric acid and hydrogen formation were carried out by mixing 100 mg cellulose or hemicellulose, and 7.80 g (3.3 mmol) H 5 PV 2 Mo 10 O 40 ·32H 2 O in 8 ml H 2 SO 4 . At room temperature, this is a slurry but on heating a clear solution is obtained. The reaction was carried out at 70 °C for 5 h under N 2 . CO and CO 2 were analysed as described above. H 2 was formed electrochemically using a platinum gauze, 25–30% oxidation at 0.6 V and the remainder at 0.2 V. H 2 was quantified by GC-TCD using a GowMac instrument with a 20′ × 1/8″ stainless steel column packed with molecular Sieve 5 Å in series with a 4′ × 1/8″ stainless steel column packed with HayeSep T. The carrier gas was Ar, column T =120 °C. Retention time was 10.0 min. Similar anaerobic reactions of cellulose in various acid solvents were carried out by mixing 100 mg cellulose and 7.80 g (3.3 mmol) H 5 PV 2 Mo 10 O 40 ·32H 2 O in 8 ml solvent. Reactions were performed under N 2 . The results are summarized in Supplementary Table 2 . Anaerobic oxidation of 13 C labelled D -glucose isomers by H 5 PV 2 Mo 10 O 40 in H 2 SO 4 were carried out by dissolving 10 mg (0.056 mmol) D -glucose ( 13 C 12 C 5 H 12 O 6 ) and 0.78 g (0.33 mmol) H 5 PV 2 Mo 10 O 40 in 98% H 2 SO 4 and the reaction mixture was heated for 5 h at 70 °C under N 2 . The relative amounts of 13 CO and 13 CO 2 were measured by GC–mass spectrometry. Cyclic voltammetry experiments Cyclic voltammetry experiments were performed using a potentiostat (CHI660A) connected to a personal computer. The measurements were performed in a three-electrode cell configuration consisting of (i) Platinum gauze (working electrode), (ii) a Pt wire (counter electrode), and (iii) Pt (a reference electrode). The experiments were performed at room temperature. The scan rate was 200 mV s −1 . The observed change in the cyclic voltammetry curve is due to the oxidation of Mo (V) to Mo (VI) before V (IV) to V (V). From our pervious studies, it is known that on reduction of H 5 PV 2 Mo 10 O 40 , vanadium atoms can be both incorporated within the polyoxometalate framework and supported as a vanayl-like cation on the polyoxmetalate surface [31] . Such different species may have different oxidation potentials. Titration with KMnO 4 The concentrations of fresh KMnO 4 solutions were determined by volumetric titration with standard oxalic acid solutions. The reduced polyoxometalate solutions were titrated volumetrically using the disappearance of the peak of the reduced polyoxometalate at 750 nm as indicator. The titrations go clearly to Mn(II). How to cite this article: Sarma, B. B. and Neumann, R. Polyoxometalate-mediated electron transfer–oxygen transfer oxidation of cellulose and hemicellulose to synthesis gas. Nat. Commun. 5:4621 doi: 10.1038/ncomms5621 (2014).